Groundwater–surface water mixing shifts ecological assembly processes and stimulates organic carbon turnover Environmental transitions often result in resource mixtures that overcome limitations to microbial metabolism, resulting in biogeochemical hotspots and moments. Riverine systems, where groundwater mixes with surface water (the hyporheic zone), are spatially complex and temporally dynamic, making development of predictive models challenging. Spatial and temporal variations in hyporheic zone microbial communities are a key, but understudied, component of riverine biogeochemical function. Here, to investigate the coupling among groundwater–surface water mixing, microbial communities and biogeochemistry, we apply ecological theory, aqueous biogeochemistry, DNA sequencing and ultra-high-resolution organic carbon profiling to field samples collected across times and locations representing a broad range of mixing conditions. Our results indicate that groundwater–surface water mixing in the hyporheic zone stimulates heterotrophic respiration, alters organic carbon composition, causes ecological processes to shift from stochastic to deterministic and is associated with elevated abundances of microbial taxa that may degrade a broad suite of organic compounds. Understanding the processes that underlie places and times of elevated biogeochemical activity is needed to construct predictive models of elemental cycling and contaminant fate and transport under future environmental scenarios. Without the knowledge of governing processes, predictions are unlikely to be accurate, owing to emergent properties that arise through the behaviour of complex systems [1] . Environmental transition zones often exhibit elevated rates of biogeochemical activity due to the mixing of complementary electron donors and terminal electron acceptors [2] , [3] , [4] . The hyporheic zone is a classic transition zone [5] , [6] , [7] important to the functioning of lotic systems [8] , [9] , [10] , [11] , [12] , [13] , [14] , where biogeochemical activity can be locally elevated during times of groundwater–surface water mixing [15] , [16] , [17] . Shifts in the hyporheic zone microbial communities are a key, but understudied, component of hydrologic mixing-induced increases in biogeochemical reaction rates. Hyporheic zone microbial ecology has primarily been studied indirectly by characterizing spatiotemporal patterns in electron donors, terminal electron acceptors and microbial biomass or activity [4] , [18] , [19] , [20] . Although connections have been made between the community composition and metabolic function of hyporheic zone microbial communities [21] , there are few studies that directly investigate hyporheic zone microbial composition [8] , [22] . This represents a significant knowledge gap, especially considering that up to 96% of lotic ecosystem respiration occurs within the hyporheic zone [12] and up to 95% of hyporheic zone respiration is microbial [23] . Although few in number, studies that directly evaluate hyporheic zone microbial communities have made important progress, revealing significant influences of sediment porosity [21] , temporal variation in physicochemical conditions [24] , [25] , [26] , heavy metal contamination [27] , [28] , [29] , groundwater–surface water exchange [30] and dissolved organic carbon composition [31] . Temporal fluctuations in river stage cause variation in the degree of groundwater–surface water mixing [32] , [33] , which in turn changes the resource environment experienced by hyporheic zone microbial communities. River stage fluctuations are therefore likely to have an indirect impact on hyporheic zone microbial community composition, mediated through changes in electron donor and/or terminal electron acceptor profiles. Although outside the spatial domain traditionally considered the hyporheic zone, Lin et al . [34] provide evidence consistent with this hypothesis, revealing significant changes in community composition associated with the intrusion of surface water into a subsurface aquifer. Stegen et al . [35] further showed that these changes in composition were due to intrusion-driven shifts in ecological selection pressures. These studies did not sample surface water or evaluate changes in the resource environment, making it difficult to understand linkages among groundwater–surface water mixing, biogeochemical conditions and community composition. Iribar et al . [36] also sampled across groundwater–surface water mixing conditions in the hyporheic zone, but did not relate changes in mixing to changes in microbial community composition. Sliva and Williams [37] used a field manipulation to study the connection between groundwater–surface water exchange and microbial composition, but found equivocal patterns due to methodological limitations. Here we evaluate the hypothesis that changes in groundwater–surface water mixing drive a coupled response in hyporheic zone biogeochemistry and microbial community composition due to shifting ecological selection pressures tied to the resource environment. To do so, we take advantage of short-term fluctuations in river stage that cause broad changes in the degree of groundwater–surface water mixing—and thus resource environment—within the Columbia River hyporheic zone and link the resulting hyporheic zone dynamics to system end members (surface water and groundwater). Although longer-term stage fluctuations are clearly important, we focus on short-term fluctuations to isolate the impacts of shifts in groundwater–surface water mixing; longer-term (for example, seasonal) sampling may confound changes in mixing with changes in other environmental variables (for example, temperature). Our analyses also leverage and combine next-generation DNA sequencing, ultra-high-resolution organic carbon profiling and ecological theory to track microbial community dynamics and reveal underlying drivers of change. We show that groundwater–surface water mixing shifts the coupled microbiome-biogeochemical system from a mixing-driven system characterized by stochastic ecological processes to a system with elevated biogeochemical rates and deterministic ecological processes. Hydrologic mixing and stimulated respiration A sampling scheme was employed adjacent to and within the Columbia River ( Fig. 1 ), to capture a range of river-stage conditions across ∼ 1 week. Although large, long-term fluctuations in river stage ( Fig. 2a ) are principally driven by snowpack melt and runoff across the Columbia River watershed, short-term fluctuations ( Fig. 2b ) are caused by up-river flow regulation at the Priest Rapids dam. Sampling across different river-stage conditions and across different spatial locations (vertically and horizontally distributed; Fig. 1 ) translated into a range of groundwater–surface water mixing conditions in the hyporheic zone as shown by substantial variation in Cl − concentration within hyporheic zone samples ( Fig. 3 ); Cl − concentration was used as a conservative tracer. The three non-conservative (that is, reactive) analytes showed remarkable differences between groundwater and surface water, which allowed for evaluations of mixing-model deviations ( Fig. 3 ); reactive analytes included non-purgable organic carbon (NPOC), dissolved inorganic carbon (DIC) and nitrate. Specific conductance—an alternative tracer of groundwater–surface water mixing conditions [38] —was logged in river water and groundwater wells. The relatively high and stable specific conductance values in groundwater wells—combined with low and stable values in the river—during the sampling period ( Supplementary Fig. 1 ) provide evidence that water sampled from groundwater wells and from the river represented distinct end members. 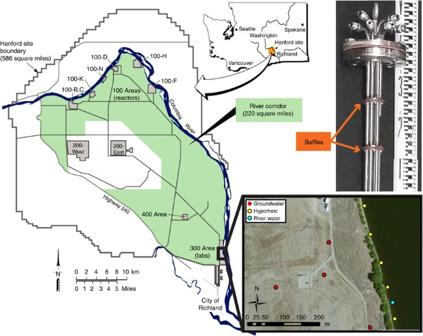Figure 1: Sampling locations and infrastructure. Map showing sampling locations in the Hanford 300 Area. Also displayed is the top 30 cm of the multi-level sampling device used to sample riverbed piezometers; baffles separating vertical zones are noted; tubes for water collection were terminated within each vertical interval. Figure 1: Sampling locations and infrastructure. Map showing sampling locations in the Hanford 300 Area. Also displayed is the top 30 cm of the multi-level sampling device used to sample riverbed piezometers; baffles separating vertical zones are noted; tubes for water collection were terminated within each vertical interval. 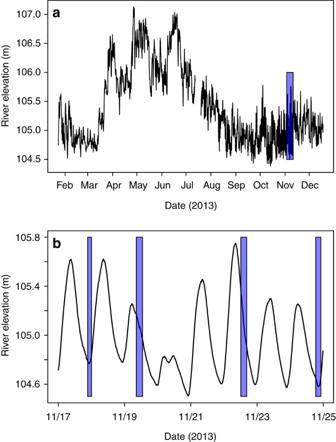Figure 2: Stage dynamics of the Columbia River and sampling intervals. (a) River stage dynamics across 2013 with the date range of sampling indicated by the overlaid rectangle. (b) River stage dynamics during the sampling period with hourly ranges of sampling indicated by the overlaid rectangles. Full size image Figure 2: Stage dynamics of the Columbia River and sampling intervals. ( a ) River stage dynamics across 2013 with the date range of sampling indicated by the overlaid rectangle. ( b ) River stage dynamics during the sampling period with hourly ranges of sampling indicated by the overlaid rectangles. 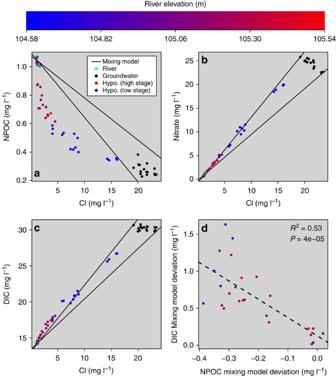Figure 3: Solutes and associated mixing models. (a–c) Dissolved solutes as a function Cl−concentration with mixing model expectations indicated by solid lines. DIC, dissolved inorganic carbon; NPOC, non-purgable organic carbon. (d) Deviation from the upper/steeper DIC mixing model as a function of the deviation from the lower/steeper NPOC mixing model. To focus on positive DIC deviations, data points were restricted to Cl−<7 mg l−1. Linear model (dashed line) statistics are provided. In all panels, river stage at the time of sample collection in the hyporheic zone is indicated by a gradient from blue (low river stage) to red (high river stage); values corresponding to colours are provided in the colour bar. Full size image Figure 3: Solutes and associated mixing models. ( a – c ) Dissolved solutes as a function Cl − concentration with mixing model expectations indicated by solid lines. DIC, dissolved inorganic carbon; NPOC, non-purgable organic carbon. ( d ) Deviation from the upper/steeper DIC mixing model as a function of the deviation from the lower/steeper NPOC mixing model. To focus on positive DIC deviations, data points were restricted to Cl − <7 mg l −1 . Linear model (dashed line) statistics are provided. In all panels, river stage at the time of sample collection in the hyporheic zone is indicated by a gradient from blue (low river stage) to red (high river stage); values corresponding to colours are provided in the colour bar. Full size image Consistent with previous studies [4] , [20] , we observed patterns in aqueous biogeochemistry that suggested elevated microbial metabolism in response to surface water intrusion into the hyporheic zone. Two groundwater–surface water mixing models were generated for each reactive analyte, revealing a region of concentrations consistent with mixing; NPOC ( Fig. 3a ) and DIC ( Fig. 3b ) concentrations commonly fell outside this space, whereas nitrate ( Fig. 3c ) concentrations did not. Positive DIC deviations were, however, only found below a Cl − concentration of ∼ 7 mg l −1 . NPOC concentrations appeared to be a single continuous function of Cl − concentrations ( Fig. 3a ), which suggests relatively consistent quality of labile carbon entering the hyporheic zone across the week of sampling; a significant decline in quality would have shifted NPOC concentrations to values more consistent with the mixing model expectation. Taken alone, the loss of NPOC—relative to the mixing expectation—could be interpreted as a signal of either enhanced microbial metabolism of organic carbon or sorption onto hyporheic zone sediments. Enhanced microbial heterotrophic respiration could increase DIC by increasing the rate of CO 2 production, whereby positive deviations would be expected from the DIC mixing model. Furthermore, assuming that the magnitude of the NPOC deviation indicates the degree to which respiration is enhanced, increasingly negative NPOC deviations would be associated with increasingly positive DIC deviations. This is indeed the pattern observed ( Fig. 3d ) and, in turn, our analyses are consistent with the hypothesis that the intrusion of surface water transports labile organic carbon into the hyporheic zone that, in turn, stimulates microbial respiration [20] , [39] . It is important to note that there is a larger DIC increase than expected from the magnitude of NPOC loss (that is, the stoichiometry is not 1:1) ( Fig. 3d ). Two factors that may contribute to the excess DIC are calcite dissolution and organic carbon ‘priming’; a recent simulation study [40] of our field system revealed that intrusion of river water into the hyporheic zone can lead to calcite dissolution and, in turn, elevated DIC; priming [41] could occur if dissolved organic carbon transported to the hyporheic zone stimulated decomposition of sediment-bound organic carbon, thereby elevating DIC. Future work that leverages isotopic signatures of abiotic and biotic sources of DIC should enable evaluation of these hypotheses. Our results indicate that the transported labile carbon is dissolved—as opposed to particulate—given that particulate organic carbon (POC) was highest in the river and did not vary significantly between the hyporheic zone and groundwater ( Supplementary Fig. 2 ). These patterns are consistent with previous work showing that POC is retained in surface sediments via filtration, thereby limiting its transport into the hyporheic zone [42] , [43] . We did observe greater variation in hyporheic zone POC concentration—relative to groundwater ( Supplementary Fig. 2 )—and the cell density of planktonic organisms was found to increase with hyporheic zone POC ( Supplementary Fig. 3 ); however, inclusion of POC from all water sources resulted in this relationship becoming nonsignificant ( P >0.05). Although the POC-cell density relationship in the hyporheic zone was relatively weak ( R 2 =0.32), it suggests that there may be times and/or places within the hyporheic zone where microbial growth due to elevated POC penetration resulted in higher biomass. Residence time of carbon-rich water in the hyporheic zone influences metabolic pathways used by hyporheic zone microbial communities [44] , [45] ; longer residence times can be associated with elevated nitrate reduction [45] due to localized depletion of O 2 (that is, anaerobic microsites) [46] , [47] , [48] . Although we do not have estimates of surface water residence time, it was probably short due to the rapid rise and fall in river elevation across the sampling timeframe ( Fig. 2b ). This is supported by previous investigations in the study system showing that—during river-stage dynamics similar to those sampled here—the direction (and magnitude) of water flux changes on a 12-h time scale due to the 12-h cycle of high/low river stage [38] . Combining estimated flux rates from Fritz and Arntzen [38] —maximum influx of river water was 0.4 l m −2 min −1 —with porosity of the hyporheic zone alluvium (0.18; ref. 49 ) provides an estimated maximum water velocity of ∼ 1.5 m per 12 h, with the vast majority of velocities across a 12-h period much slower than this [38] . The regular reversal of the hydrologic gradient—and low river elevation minima during the sampling period ( Fig. 2 )—suggests that the residence time of river water in the hyporheic zone was on the order of 1 day. The consistency between hyporheic zone concentrations and mixing model expectations are therefore not surprising. It is likely that denitrification was not stimulated by surface water intrusion, because modest residence times, high O 2 concentrations in intruding surface water and low NPOC concentrations collectively resulted in severe reaction-rate limitation [50] . In addition, significant O 2 can be maintained in the hyporheic zone—and therefore inhibit denitrification [2] —under organic carbon concentrations similar to those observed here, even when residence times are two orders of magnitude longer than estimated here [51] . We further note that these conditions (high O 2 and low NPOC) may be more conductive to nitrification than denitrification [2] , [52] , which could lead to a positive deviation from the mixing model, but such a pattern was not apparent ( Fig. 3 ). The significant loss of NPOC during times of surface water intrusion suggests that changes in the organic carbon profile may drive shifts in microbial community composition [31] . If there is such an effect, it could be mediated by the quantity and/or composition of organic carbon. To distinguish between these possibilities, we complemented the NPOC quantification with ultra-high-resolution carbon profiling, using Fourier transform ion cyclotron resonance mass spectrometry (FT-ICR MS). Shifts in organic carbon and microbial community composition Considering all water sources together, the composition of organic carbon—as characterized by FT-ICR MS—varied significantly ( P =0.001) with changes in NPOC concentration ( Fig. 4a ) and this relationship was stronger ( r =0.66) than one based on changes in Cl − concentration ( r =0.55). In addition, the median mass-to-charge ratio within a given sample varied significantly across water sources ( P <0.05), with larger values in groundwater ( Fig. 4b ). Low-molecular-weight organic carbon in the hyporheic zone, relative to groundwater, is consistent with increased microbial activity [53] . This further supports our inference that labile organic carbon—transported by intruding river water—stimulates microbial respiration in the hyporheic zone. 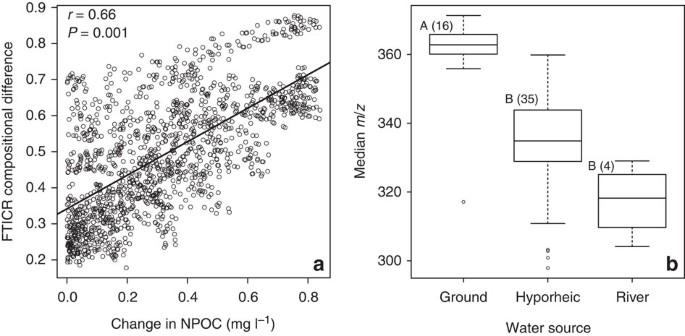Figure 4: Variation in FT–ICR MS-based dissolved organic carbon composition. (a) Change in carbon composition—measured as Sorensen dissimilarity, bounded between 0 and 1—as a function of change in NPOC concentration. The solid line indicates the regression model and associated Mantel test statistics are provided. (b) Box plots summarizing distributions of mass-to-charge ratios (m/z) across different water sources. Different letters indicate statistically significant differences (P<0.05) by a Kruskal–Wallis test and values in parantheses are the number of samples in each group. Figure 4: Variation in FT–ICR MS-based dissolved organic carbon composition. ( a ) Change in carbon composition—measured as Sorensen dissimilarity, bounded between 0 and 1—as a function of change in NPOC concentration. The solid line indicates the regression model and associated Mantel test statistics are provided. ( b ) Box plots summarizing distributions of mass-to-charge ratios ( m / z ) across different water sources. Different letters indicate statistically significant differences ( P <0.05) by a Kruskal–Wallis test and values in parantheses are the number of samples in each group. Full size image Although organic carbon composition varied significantly with changes in NPOC concentration and water source ( Fig. 4 ), it was not strongly related to microbial community composition (see below). However, we consider this evaluation preliminary, because our use of the FT-ICR MS data was limited to the presence/absence of unique m / z peaks. This approach does not capture important shifts in the relative abundance of labile carbon species, which may obscure the relationship between carbon composition and microbial community composition. We consider this probable given that previous work has shown a strong influence of carbon composition over hyporheic zone community composition [31] . Preliminary data exploration indicated that changes in community composition were most strongly related to shifts in Cl − and NPOC concentrations, with weaker relationships observed for changes in FT-ICR MS-based carbon composition and changes in temperature. In addition, the number of unique operational taxonomic units (OTUs) increased significantly with Cl − concentration and declined significantly with NPOC concentration ( Supplementary Fig. 4 ); these relationships were effectively equivalent in terms of variation explained ( R 2 ≈0.45 and P <<0.0001 for both). In turn, we focus on microbial composition as related to Cl − and NPOC concentrations. Relating three metrics of community turnover—Bray–Curtis, β-mean nearest taxon distance (βMNTD) and β-nearest taxon index (βNTI)—to shifts in Cl − and NPOC concentrations revealed important influences of both groundwater–surface water mixing and changes in the resource environment. The Bray–Curtis and βMNTD metrics respectively quantify turnover in the relative abundances of OTUs and in community phylogenetic structure. These are ‘raw’ metrics and do not, by themselves, carry information about the ecological processes that govern community turnover [54] , [55] , [56] . That is, variation in the magnitudes of these two metrics can be driven by stochastic ecological processes such as organismal dispersal and more deterministic ecological processes associated with environmental or habitat selection. Bray–Curtis was nonlinearly related to changes in Cl − concentration ( Fig. 5a ), but a weak relationship was observed with respect to changes in NPOC concentration ( Fig. 5b ). βMNTD was significantly ( P =0.001 for both) related to changes in both Cl − and NPOC concentrations ( Fig. 5c,d ); the relationship with Cl − ( r =0.70) was stronger than with NPOC ( r =0.52). Although a change in NPOC concentration probably reflects alteration of the resource environment, a change in Cl − concentration arises due to the transport of surface water into (or out of) the subsurface domain. The Bray–Curtis and βMNTD patterns therefore suggest that the transport of surface water may directly influence OTU relative abundances and community phylogenetic structure. One parsimonious interpretation is that the transport of surface water into the subsurface enhances organismal dispersal across system compartments (that is, from surface water to the hyporheic zone to the broader aquifer). Importantly, this indicates that organismal dispersal can influence community composition, but it does not rule out a strong influence of the resource environment. An alternative interpretation is that uranium contamination—which closely tracks groundwater–surface water mixing conditions in the study system [38] —may influence community composition. Konopka et al . [57] showed, however, that microbial activity in the study system is not altered by prevailing uranium concentrations due to formation of carbonate uranyl complexes. 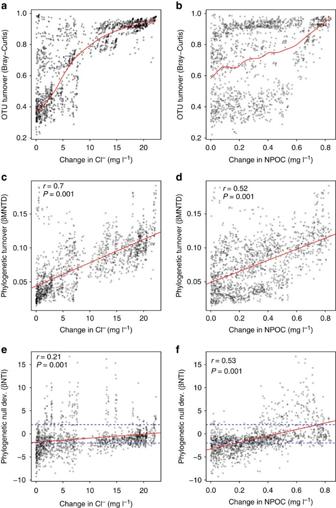Figure 5: Turnover in microbial community composition. Microbial community turnover in terms of composition (a,b), phylogeny (c,d) and phylogenetic null model deviation (e,f). Turnover metrics are related to either changes in Cl−(a,c,e) or changes in NPOC (b,d,f). Solid red lines indicate a nonlinear spline fit (a,b) or linear models (c–f); dashed blue lines (e,f) indicate null model deviation significance thresholds; values above +2 or below −2 are considered significant. Mantel test statistics are provided. Figure 5: Turnover in microbial community composition. Microbial community turnover in terms of composition ( a , b ), phylogeny ( c , d ) and phylogenetic null model deviation ( e , f ). Turnover metrics are related to either changes in Cl − ( a , c , e ) or changes in NPOC ( b , d , f ). Solid red lines indicate a nonlinear spline fit ( a , b ) or linear models ( c – f ); dashed blue lines ( e , f ) indicate null model deviation significance thresholds; values above +2 or below −2 are considered significant. Mantel test statistics are provided. Full size image Ecological processes The βNTI metric provides deeper insights into the potential role of the resource environment, because variation in the magnitude of βNTI is driven primarily by variation in the selective environment and, to a much lesser extent, by organismal dispersal [56] . The reason is that βNTI is based on a null model that factors out influences of stochastic ecological processes such as organismal dispersal and ecological drift. In turn, if the resource environment does have an impact on the structure of hyporheic zone microbial communities, we expect three patterns: (i) a significant relationship between βNTI and changes in NPOC; (ii) this relationship should be stronger than the relationship between βNTI and changes in Cl − ; and (iii) with small changes in NPOC, βNTI values should be below −2 and βNTI should increase to above +2 with increasingly large NPOC changes. The reason for (iii) is that small changes in NPOC indicate there is a consistent resource environment and βNTI<−2 indicates that a consistent selective environment causes high similarity in community composition. Likewise, larger changes in NPOC indicate there is a large change in the resource environment and βNTI>+2 indicates that a change in the selective environment causes a significant shift in community composition [56] , [58] . As shown in Fig. 5e,f , βNTI was significantly ( P =0.001 for both) related to changes in both Cl − and NPOC concentrations ( Fig. 5e,f ); the relationship with NPOC ( r =0.53) was stronger than with Cl − ( r =0.21) and transitioned from βNTI<−2 (with small changes in NPOC) to βNTI >+2 (with large changes in NPOC) ( Fig. 5f ). All three expectations were therefore met, which provides evidence that changes in the resource environment deterministically cause shifts in microbial community composition. It is important to recognize that these resource-based influences worked alongside influences of organismal dispersal, and that neither process dominated the system. Coupling NPOC deviations with βNTI further revealed that homogeneous ecological selection [56] , [58] , [59] emerged in places and times of mixing. More specifically, median βNTI values for a given sample were significantly ( P =0.0009, R 2 =0.19) and positively related to the deviation from the NPOC mixing model ( Fig. 6a ); this relationship was stronger when considering only hyporheic zone samples ( P =0.0001, R 2 =0.37). Median βNTI values associated with negative NPOC deviations were also significantly ( P <<0.0001) more negative than βNTI values associated with effectively no deviation ( Fig. 6b ). Negative NPOC deviations—which we equate with groundwater–surface water mixing-induced increases in microbial activity—were therefore associated with βNTI values centred near −2, which indicates a shift to a selective environment dominated by a small number of consistently imposed selective pressures (that is, homogeneous ecological selection). This aligns with experimental results of Findlay et al . [31] but contrasts sharply with microbial communities from the current study associated with no effective deviation from the NPOC mixing model; these communities were associated with βNTI values (centred near −1) consistent with stochastic ecological processes [58] . 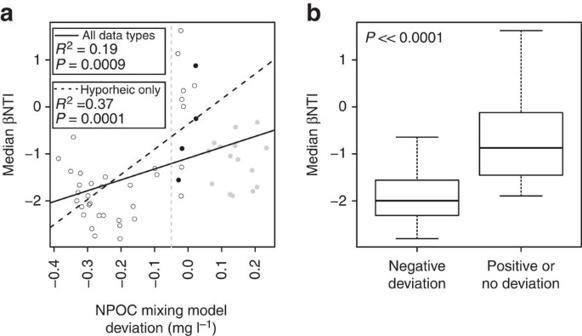Figure 6: Relationships between βNTI and mixing model deviations. (a) βNTI estimate of each community as a function of the deviation between observed and expected NPOC; the solid line indicates the regression model and statistics are provided; open, closed black and closed grey symbols indicate hyporheic, river and ground water samples, respectively.(b) Box plots summarizing distributions of median βNTI values—froma—that are or are not associated with a negative NPOC deviation; βNTI values included in the ‘negative deviation’ distribution are to the left of the dashed grey line inaand all other βNTI values are included in the ‘positive or no deviation’ distribution; the displayedP-value indicates a significant difference between distributions by a Kruskal–Wallis test. Figure 6: Relationships between βNTI and mixing model deviations. ( a ) βNTI estimate of each community as a function of the deviation between observed and expected NPOC; the solid line indicates the regression model and statistics are provided; open, closed black and closed grey symbols indicate hyporheic, river and ground water samples, respectively. (b ) Box plots summarizing distributions of median βNTI values—from a —that are or are not associated with a negative NPOC deviation; βNTI values included in the ‘negative deviation’ distribution are to the left of the dashed grey line in a and all other βNTI values are included in the ‘positive or no deviation’ distribution; the displayed P -value indicates a significant difference between distributions by a Kruskal–Wallis test. Full size image Microbial taxa connected to biogeochemical shifts To assess possible microbial drivers of NPOC consumption in the hyporheic zone, community structure within samples exhibiting different magnitudes of deviation from the NPOC mixing model were compared. To remove effects of groundwater–surface water mixing, only samples with similar Cl − concentrations were compared against each other; we did not constrain the spatial and temporal relationships between pairs of samples selected for this analysis. Six pairs of samples were compared and 11 OTUs increased in relative abundance as NPOC deviations grew larger. In some instances, significant enrichments were measured between samples (>6% relative abundance increase) ( Fig. 7 ). 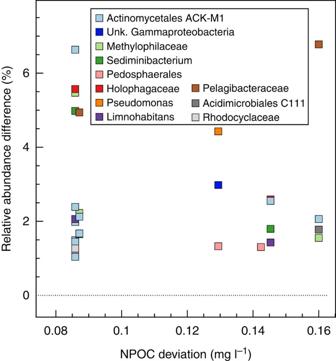Figure 7: Microbial groups exhibiting increased relative abundance in samples with greater NPOC deviation from the mixing model. Relative abundance comparisons were made between samples with similar mixing conditions. Figure 7: Microbial groups exhibiting increased relative abundance in samples with greater NPOC deviation from the mixing model. Relative abundance comparisons were made between samples with similar mixing conditions. Full size image Limitations of 16S ribosomal RNA analyses prevent species-level identifications and inferences of exact metabolic potential, but taxonomic placings may be used to broadly assess physiological roles; most broadly, microbial groups assigned to the 11 OTUs all contain heterotrophic members. OTUs affiliated with the Actinomycetales ACK-M1 lineage exhibited a particularly strong increase in relative abundance concomitant with a greater loss of NPOC, relative to the mixing model ( Fig. 7 ). Environmental strains within the Actinomycetales have been shown to contain increased numbers of ABC-type mce transporters, which may enable metabolic versatility in environments containing varied carbon substrates such as NPOC [60] . Likewise, members of the genus Limnohabitans isolated from aquatic environments have previously shown high rates of substrate uptake and the ability to grow on simple organic acids and sugars [61] . The largest relative abundance increase between two samples exhibiting the greatest NPOC deviation was for an OTU affiliated with the Pelagibacteraceae ( ∼ 7% relative abundance increase). Species within this family—members of the SAR11 cluster—are thought to be the most abundant microorganisms on Earth and recent studies have focused on the ecophysiology of a SAR11 freshwater sister group, termed LD12 (ref. 62 ). Studies have demonstrated that members of this group exhibit both a pronounced preference for uptake of glutamine and glutamate over other amino acids and higher uptake rates for these substrates relative to other freshwater community members [62] . These microorganisms also use other simple organic compounds such as acetate, glucose and fructose. Considering our results collectively, we infer that when surface water intrusion delivers labile organic carbon to the hyporheic zone, it stimulates microbial activity, but does so non-randomly through imposition of a homogeneous ecological selective environment [56] , [58] , [59] . We further infer that in places and times in which there is no (or insufficient) groundwater–surface water mixing, microbial community composition is governed principally by organismal dispersal. Evaluations of these inferences are needed beyond our study system, the timespan it was sampled and suspended microbes. Biogeochemical activity is often enhanced at environmental transitions due to reciprocal provisioning of resources that limit activity in one environment but are abundant in the other [3] . The hyporheic zone is a classic example of this dynamic [15] and here we aimed to evaluate coupled dynamics between the biogeochemical environment and microbial composition, in response to changes in groundwater–surface water mixing within the hyporheic zone. Our results suggest that—across the spatial and temporal scales studied here—microbial communities within groundwater or surface water are governed by stochastic ecological processes, but that surface water intrusion into the hyporheic zone delivers labile organic carbon that stimulates microbial respiration and causes (ecologically) deterministic shifts in microbial community composition. We have revealed a collection of field-scale patterns that are consistent with a strong impact of surface water intrusion on hyporheic zone microbiomes and biogeochemical function. There are numerous mechanisms underlying these coupled dynamics that will require additional investigation. To guide future efforts and connect our study to a broader range of systems, we collate the patterns observed here into a conceptual model ( Fig. 8 ). It is important to note that the conceptual model developed below is speculative and represents a collection of hypotheses that emerge from our results; it is intended to be a point of departure for future work. The conceptual model is most relevant to systems that transition between saturated and unsaturated conditions, such as sections of rivers that are influenced by dam operations and/or tides. We frame the conceptual model around a key question: what is the source (or sources) of labile organic carbon that is transported by surface water and why is it not consumed before entering the hyporheic zone? 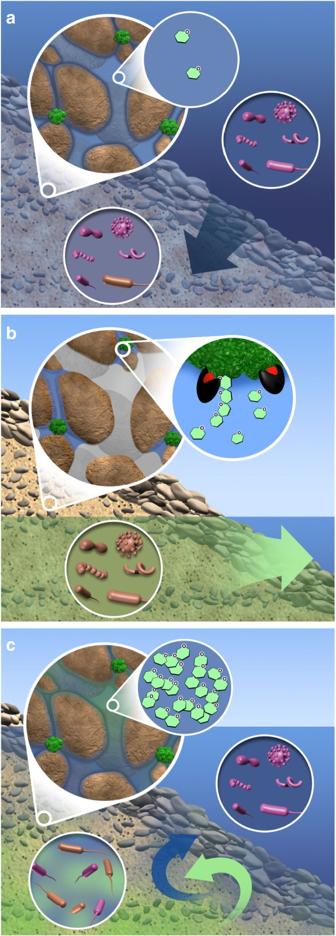Figure 8: Conceptual depiction of hypothesized dynamics in the hyporheic zone driven by changes in river stage. (a) At high stage, the hyporheic zone is inundated with river water (dark blue arrow). Unattached microbial communities in the river and hyporheic zone are governed by stochastic ecological processes whereby a broad range of microbial taxa are present (visualized as different cell shapes); purple and brown cells represent river-derived and groundwater-derived microbial taxa, respectively. Well-connected pore channels and active microbial communities limit the accumulation of labile organic carbon (visualized as saccharide molecules) in pore channels. (b) At low river stage, the hyporheic zone is dominated by groundwater discharge (green arrow) and unattached microbial communities are governed by stochastic ecological processes. Large interconnected pores drain—but smaller pores do not—following the decline in river stage. Extracellular enzymes (black and red) continue to degrade POC into labile organic carbon; however, owing to unsaturated conditions, highly tortuous paths with long diffusion times delay the transport of labile carbon to microbial cells. The result is accumulation of labile carbon within microsites and along tortuous paths. (c) A rise in river stage causes groundwater–surface water mixing that leads to deterministic ecological processes that select for microbial taxa with particular ecological traits (indicated by a single cell shape in the hyporheic zone). The re-saturation of sediments disperses accumulated labile carbon into large pores, thereby decreasing transport times to microbial cells and, in turn, stimulating heterotrophic respiration. Figure 8: Conceptual depiction of hypothesized dynamics in the hyporheic zone driven by changes in river stage. ( a ) At high stage, the hyporheic zone is inundated with river water (dark blue arrow). Unattached microbial communities in the river and hyporheic zone are governed by stochastic ecological processes whereby a broad range of microbial taxa are present (visualized as different cell shapes); purple and brown cells represent river-derived and groundwater-derived microbial taxa, respectively. Well-connected pore channels and active microbial communities limit the accumulation of labile organic carbon (visualized as saccharide molecules) in pore channels. ( b ) At low river stage, the hyporheic zone is dominated by groundwater discharge (green arrow) and unattached microbial communities are governed by stochastic ecological processes. Large interconnected pores drain—but smaller pores do not—following the decline in river stage. Extracellular enzymes (black and red) continue to degrade POC into labile organic carbon; however, owing to unsaturated conditions, highly tortuous paths with long diffusion times delay the transport of labile carbon to microbial cells. The result is accumulation of labile carbon within microsites and along tortuous paths. ( c ) A rise in river stage causes groundwater–surface water mixing that leads to deterministic ecological processes that select for microbial taxa with particular ecological traits (indicated by a single cell shape in the hyporheic zone). The re-saturation of sediments disperses accumulated labile carbon into large pores, thereby decreasing transport times to microbial cells and, in turn, stimulating heterotrophic respiration. Full size image To develop a potential answer to this question, we note that the rise and fall of river stage results in saturated/unsaturated dynamics in near-surface hyporheic zone sediments that are similar to—although not as extreme as—wetting/drying dynamics in semi-arid soils. It is well known that rewetting of semi-arid soils causes a rapid increase in CO 2 emissions (that is, the ‘Birch Effect’) [63] , [64] , [65] . Mechanisms underlying this phenomenon probably vary across systems, but are grouped into two categories [66] : (i) the ‘supply hypothesis’ posits that rewetting increases the supply of labile organic carbon through physical process such as aggregate dissolution and hydrologic redistribution of spatially isolated organic matter [67] ; and (ii) the ‘stress hypothesis’ posits that rewetting causes drought adapted microorganisms to either lyse due to rapid increases in turgor pressure or to rapidly excrete labile osmolytes to avoid lysis [68] , [69] . The stress and supply hypotheses contain multiple potential mechanisms, but considering details of our study system allows refinement. Given the relatively rapid rise and fall of river stage ( Fig. 2b ), sediments would not have desiccated such that hyporheic zone microbes would not have been osmotically stressed; we thus reject the stress hypothesis as an explanation for dynamics in our study system. Aggregate dissolution—and the associated release of occulated organic matter—is one mechanism underlying the supply hypothesis [66] , but is unlikely in light of the repeated saturated/unsaturated cycles and the consistent biogeochemical response observed here; repeated high/low moisture cycles select for stable aggregates [70] and aggregate dissolution should result in a progressively diminished biogeochemical response [71] , yet hyporheic zone NPOC concentration can be described as one continuous function of groundwater–surface water mixing conditions. We suggest that a more probable scenario is a combination of (i) physical isolation of sediment-associated microorganisms—the primary drivers of organic carbon cycling, but not directly studied here—from organic matter following the transition from advective to diffusion-based transport; a decline in river stage results in unsaturated conditions and, in turn, diffusion-based transport; and (ii) the rapid transport of dissolved organic carbon through the hyporheic zone as river stage rises ( Fig. 8 ). We specifically hypothesize that extracellular enzymes continue to degrade large organic molecules—supplied as POC—in locations that microorganisms cannot access (temporarily) due to diffusion-based transport during low river stage (that is, during times of desaturation). Labile organic carbon would, in this case, accumulate in isolated microsites during low river stage and—following an increase in river stage—subsequently be dispersed and carried into the hyporheic zone at a rate that exceeds the ability of recently re-saturated communities to metabolize it. This mechanism is consistent with models that indicate accumulation of labile carbon during dry periods [72] , [73] and observations that enzyme activities are less impacted by soil moisture than is microbial biomass [74] , suggesting continued enzymatic activity in times of reduced microbial activity [75] . The patterns observed here suggest that transported labile carbon may be progressively consumed along hyporheic zone flow paths [20] , [39] —thereby stimulating microbial activity—and may also select for particular microbial taxa that can efficiently use the transported substrates ( Fig. 8 ). Extending these concepts leads to an additional hypothesis: longer times between surface water inundations lead to greater accumulation of labile carbon within microsites, which is consistent with observations in soil systems [71] . If this is true, then less frequent (and large) increases in river stage may disperse and transport larger quantities of labile organic carbon into the hyporheic zone and, in turn, may cause greater enhancement of microbial activity. Higher rates of microbial respiration can generate anaerobic microsites [47] and promote removal and/or immobilization of nitrate and other redox-sensitive contaminants [44] . This suggests an important link between climate-change-driven shifts in watershed hydrology and the rates of elemental cycling and contaminant dynamics. If large pulses of water associated with Spring-time snowpack melt (for example, Fig. 2a ) are diminished by warmer winter temperatures, microbial respiration rates may be too low to deplete O 2 , therefore having a significant impact on contaminant dynamics. To rigorously evaluate the potential for such outcomes (for example, through predictive hydro-biogeochemical models), the hypotheses that constitute our proposed conceptual model (see Fig. 8 ) will need to be directly tested and refined. Field sampling Samples were collected from the Columbia River, its hyporheic zone (sediment porosity of ∼ 0.18 and hydraulic conductivity of ∼ 1–4 m per day, from ref. 49 ) and the adjacent unconfined aquifer underlying the Hanford 300 Area (sediment porosity of ∼ 0.20 and hydraulic conductivity of ∼ 7,000–8,000 m per day, from ref. 49 ) ( Fig. 1 ). To capture a broad range of groundwater–surface water mixing conditions, we targeted different river stages across four time intervals in November 2013; river stage was monitored ∼ 300 m downstream of our field sampling locations using a pressure transducer coupled to a CR1000 datalogger (Campbell Scientific Inc., for both). The range of sampled mixing conditions was further enhanced by taking advantage of spatial heterogeneity within the hyporheic zone; the hyporheic zone was sampled at multiple depths at each of five locations ( Fig. 1 ) using a custom-built multi-level sampling device ( Fig. 1 ) installed within fully screened stainless steel piezometers; 1.2 m screen length and 5.25 cm inside diameter (MAAS Midwest, Huntley, IL). The most Northern piezometer ( Fig. 1 ) was sampled within the depth intervals of ∼ 1–11 and ∼ 41–51 cm (it could not be installed to full depth) and the other four piezometers were sampled within the depth intervals of ∼ 10–20 and 110–120 cm. The five sampled piezometers were not meant to be replicates, but were instead assumed to capture different physical features of the hyporheic zone such that sampling across them provided access to a broader range of mixing conditions. Groundwater was sampled from four wells screened across the top of the subsurface aquifer ( Fig. 1 ) and river water was sampled near the piezometers. Water from the hyporheic zone and the river were sampled using a peristaltic pump and the subsurface aquifer was sampled using submersible pumps; all systems were purged—the equivalent of at least three volumes—before sample collection. At each location and depth, pumped water passed through 0.22 μm polyethersulfone Sterivex filters (Millipore Co., Billerica, MA) for ∼ 30 min or until 10 l had passed through a filter, whichever came first; sampled volume ranged from 1.33 to 10 l. Sampling time was constrained instead of sampled volume because of the dynamic nature of groundwater–surface water mixing conditions within the hyporheic zone of our system; changing the filtration time across samples to achieve a consistent volume could have resulted in some filters collecting microbes across larger ranges of mixing conditions. In addition, we note that no relationships emerged in the hyporheic zone between filtered volume and (i) the concentrations of aqueous analytes (NPOC, DIC, Cl − and ; R 2 <0.05 for all) or (ii) the microbial community turnover metrics (Bray–Curtis, βMNTD and βNTI; Mantel r ≤0.1 for all). Filters were collected, frozen on dry ice in the field and stored at −80 o C. Sterivex-filtered water was used to collect samples for water chemistry. Samples for anions and dissolved organic and inorganic carbon were collected into pre-cleaned 40 ml glass vials (Thermo Scientific), stored at 4 °C and split for ion chromatographic and carbon analysis in the lab. Samples for organic carbon profiling were also taken in 40 ml glass vials and frozen at −20 °C. Cation samples were taken in 15 ml polypropylene tubes (Becton Dickinson Co., Franklin, NJ) pre-acidified with 0.1 ml, 70% HNO 3 and stored at 4 °C. Handheld meters were used to measure water temperature and conductivity (Ultrameter II, Myron L Co., Carlsbad, CA). Simultaneously, unfiltered water was preserved in glutaraldehyde (1% final) for cell counts in 15 ml polypropylene tubes (Corning Inc. Corning, NY) and stored at 4 °C, and was separately filtered through pre-combusted 47 mm glass-fibre filters (Whatman, GE Healthcare, UK) for quantification of POC. Water volume filtered for POC was quantified, with a target of 10 l, and filters were stored at −20 °C in plastic petri dishes. Analytical methods POC samples were removed from the freezer and air dried in a biological safety cabinet, then cut into pieces to fit into a folded cup of 40 × 40 mm silver foil (Elementar Co., Germany). Cut POC filters were acidified dropwise with 1.2 N HCl, to remove inorganic carbon, and dried in a fume hood. POC filters in silver foil were wrapped in 50 × 50 mm squares of pure tin foil (Elemental Microanalysis, UK) and compressed, to remove air, with a manual pressing tool (Elementar Co.). POC samples were analysed for C, N & S using an Elementar vario EL cube. DIC and NPOC were determined with a Shimadzu combustion carbon analyser TOC-Vcsh with ASI-V auto sampler. The DIC was determined by injection into 25% phosphoric acid at ambient temperature. Inorganic carbon standards were made from sodium bicarbonate and sodium carbonate solids (Nacalia Tesque). The calibration range for the DIC determinations was from 0.35 to 40 mg l −1 as C and measurement error was 0.5%. The NPOC was determined by acidification of the sample with 2 N HCl (Optima, Fisher) with a 5-min sparging time to remove DIC. The sample was then injected into the furnace set to 680 °C. The organic carbon standards were made from potassium hydrogen phthalate solid (Nacalia Tesque). The calibration range for the NPOC determinations was from 0.35 to 3.5 mg l −1 as C and measurement error was 0.4%. A Dionex ICS-2000 anion chromatograph with AS40 auto sampler was used to determine and Cl − concentrations. The guard column was an IonPac AG18 guard, 4 × 50 mm (Dionex). The analytical column was an IonPac AS18, 4 × 250 mm (Dionex). The suppressor was an RFIC ASRS, 300 4-mm, self-regenerating (Dionex) and the suppressor current was set at 99 mA. A 25-min gradient method was used with 25 μl injection volumes and a 1 ml min −1 flow rate at 30 °C. KOH (22 mM) was used for the first 7 min. From 7 to 8 min, the KOH concentration increased from 22 to 40 mM. From 8 to 20 min, 40 mM KOH was used. From 20 to 25 min, the KOH concentration decreased from 40 to 22 mM. The suppressor current was set to 99 mA. Anion standards were prepared from Spex CertiPrep (Metuchen, NJ; 08840). Anion standards (1,000 mg l −1 ) were diluted for a calibration range from 0.60 to 120 p.p.m. and measurement error was 2.5% for Cl − and 1.4% for . Cell densities were estimated from glutaraldehyde-preserved samples using a BD Influx Flow Cytometer (Becton Dickinson, San Jose, CA) with 488-nm excitation from a Sapphire LP laser (Coherent Inc., Santa Clara, CA, USA) at 100 mW. Optimization and calibration of the fluorescence-activated cell sorting was performed using 3 μm Ultra Rainbow Fluorescent Particles (Spherotech, Lake Forest, IL, USA). Samples were vortexed and a 500-μl aliquot was stained with SYBR Gold (Life Technologies, Grand Island, NY) at a concentration of 1:1,000 in the dark for 10 min at room temperature; an unstained sample was acquired to determine background fluorescence. A population gate was set to count stained events and a 100-μl subsample was used to prime the sample line. When events were detected, the initial subsample was removed and a second 100-μl subsample was loaded onto the instrument and data acquisition was started; the entire sample was analysed. For normalization, the number of background events was subtracted from the number of events counted in stained subsamples. Organic carbon characterization Ultra-high-resolution characterization of dissolved organic carbon was carried out using a 15-T Bruker SolariX FT-ICR MS located at the Environmental Molecular Sciences Laboratory, a Department of Energy–Office of Biological and Environmental Research national user facility in Richland, WA. Samples were thawed overnight and then prepared by adding 0.5 ml methanol (LC/MS grade Optima, Sigma Aldrich, St Louis, MO) to 0.5 ml of sample water in an Eppendorf 96-well plate fitted with 2 ml glass sleeves. Suwannee River Fulvic Acid (SRFA) standard (International Humic Substances Society) was used as a control and injected every 15th sample, to assure instrument stability. SRFA is the most commonly used standard for characterization of organic matter and humic material, and its composition has been extensively characterized [76] , [77] , [78] , [79] . The carbon (C) content of SRFA is 52.44% (refs 76 , 77 ). SRFA samples were prepared from the International Humic Substances Society as received powder at 1 mg ml −1 in MilliQ filtered water and diluted to 2 μg ml −1 to serve as a control. Lab blanks were prepared, 50/50 LC/MS grade methanol/MilliQ filtered water (v/v) were then injected after the control, to verify no sample carryover. Samples were injected directly into the instrument using an automated custom-built system and ion accumulation time was optimized for all samples. A standard Bruker electrospray ionization source was used to generate negatively charged molecular ions. Samples were introduced to the electrospray ionization source equipped with a fused silica tube (30 μm intradermally) through an Agilent 1200 series pump (Agilent Technologies) at a flow rate of 3.0 μl min −1 . Experimental conditions were as follows: needle voltage +4.4 kV, Q1 set to 50 m / z and the heated resistively coated glass capillary operated at 180 °C. These were optimal parameters established in earlier dissolved organic carbon characterization experiments. One hundred and forty-four individual scans were averaged for each sample and internally calibrated using an organic matter homologous series separated by 14 Da (–CH 2 groups). The mass measurement accuracy was typically within 1 p.p.m. for singly charged ions across a broad m / z range (100–1,100 m / z ). The mass resolution was 350,000 at 339.112 Da. DataAnalysis software (BrukerDaltonik version 4.2) was used to convert raw spectra to list of m / z values applying Fourier transform mass spectrometry peak picker with S / N threshold set to 7 and absolute intensity threshold to the default value of 100. Change in organic carbon profile between samples was based on the shifts in the presence/absence of m / z peaks and was quantified using the Sorensen dissimilarity metric commonly used in ecological studies, to measure turnover in community composition; the distance function in the ecodist R package was used for Sorensen calculations. DNA extraction and processing For each Sterivex filter, the housing was cracked open and the filter was removed using sterile instruments. DNA was extracted using a modification of methods from Bostrom et al . [80] . Filter material was incubated at 85 o C for 15 min in lysis buffer, as defined in Bostrom et al . [80] To avoid DNA fragmentation, the solution was slowly cooled and lysozyme was added to a final concentration of 1 mg ml −1 . The resulting solution was incubated at 37 °C for 30 min. SDS was added to 1% final concentration and proteinase-K was added to 100 μl ml −1 final concentration. The resulting solution was incubated at 55 °C for ∼ 12 h. To facilitate cell lysis, samples were run through three freeze–thaw cycles using liquid N 2 followed by warming to 55 °C. The sample was then vortexed followed by isopropanol precipitation and pellet elution in TE [80] . The sample was then treated with 10 μg ml −1 RNase at 37 °C for 30 min, followed by phenol–chloroform clean-up, isopropanol precipitation and elution in TE. Extracted DNA was stored at −20 °C until shipment (on dry ice) to the sequencing facility at Argonne National Laboratory. At Argonne National Laboratory, DNA was amplified using the Earth Microbiome Project barcoded primer set, adapted for the Illumina MiSeq by adding nine extra bases in the adapter region of the forward amplification primer that support paired-end sequencing. The V4 region (515F-806R) of the 16S rRNA gene was amplified with region-specific primers that included the Illumina flowcell adapter sequences. The reverse amplification primer contained a 12-base barcode sequence that supports pooling of up to 2,167 samples in the single MiSeq lane [81] , [82] . Each 25 μl of PCR reaction contained 12 μl of MoBio PCR Water (Certified DNA-Free), 10 μl of 5 Prime HotMasterMix (1 ×), 1 μl of Forward Primer (5 μM concentration, 200 pM final), 1 μl Golay Barcode Tagged Reverse Primer (5 μM concentration, 200 pM final) and 1 μl of template DNA. The conditions for PCR were as follows: 94 °C for 3 min to denature DNA, with 35 cycles at 94 °C for 45 s, 50 °C for 60 s and 72 °C for 90 s; with a final extension of 10 min at 72 °C, to ensure complete amplification. Amplicons were quantified using PicoGreen (Invitrogen) and a plate reader. Appropriate volumes of PCR product from each sample were then pooled so that each sample was represented with an equal amount of product. This pool was cleaned using the UltraClean PCR Clean-Up Kit (MoBIO), and quantified using the Qubit (Invitrogen). After quantification, the molarity of the pool was determined and diluted to 2 nM, denatured and then diluted to a final concentration of 6.75 pM with a 10% PhiX spike for sequencing on the Illumina MiSeq. Resulting sequences were processed in QIIME 1.8.0 (ref. 83 ). First, the function split_libraries_fastq.py was used to demultiplex the fastq-formatted sequences, with a Phred [84] quality cutoff of 20. To identify chimeras the function identify_chimeric_seqs.py was used to call USEARCH v6.1 (ref. 85 ) with ‘non_chimera_retention’ set to ‘intersection.’ After removing identified chimeras (with function filter_fasta.py), the function pick_open_reference_otus.py was used to call USEARCH v6.1, pick OTUs and generate the associated phylogeny using SILVA (97% similarity, release 111) ( http://www.arb-silva.de/ ) as the reference; default parameters were used, except for the following modifications: ‘suppress_de_novo_chimera_detection’, ‘suppress_reference_chimera_detection’ and ‘derep_fullseq’ were all set to ‘True’ and ‘prefilter_percent_id’ was set to 0. All additional analyses were carried out in R ( http://cran.r-project.org/ ). OTUs identified as chloroplasts were removed and the OTU table was subsequently rarefied to the lowest number of sequences (4,899) found within an individual sample using the rrarefy function in the vegan package. OTUs that had zero abundance across all samples, following rarefaction, were removed from both the OTU table and the phylogeny using the match.phylo.data function in the picante library. The number of OTUs present in each sample (OTU richness) was enumerated as an estimate of microbial diversity. The Bray–Curtis metric was used to quantify turnover in community composition and was calculated with the distance function in the ecodist package. βMNTD was used to quantify turnover in the phylogenetic structure of communities; abundance weighted βMNTD was calculated using the comdistnt function in the picante package (see also refs 35 , 55 , 58 , 86 ). To evaluate the potential for shifts in the relative balance between stochastic and deterministic ecological processes, randomizations were used to generate a null distribution (999 randomizations) for each βMNTD estimate; βMNTD is a pairwise distance metric such that a null βMNTD distribution was generated for each pairwise community comparison. The βNTI measures the difference between observed βMNTD and the mean of the null distribution in units of standard deviations (see also refs 35 , 55 , 58 , 86 ): Statistical analyses To characterize groundwater–surface water mixing conditions within the hyporheic zone we assumed Cl − to be a conserved tracer and took advantage of large differences in Cl − concentration between groundwater and surface water. Low variation was observed within river water for Cl − and the reactive analytes of interest (that is, , NPOC and DIC), but greater variation was observed within groundwater. In turn, two linear mixing models were generated for each analyte using mean river water conditions as one end-member and extreme groundwater conditions as the other end-member; for example, one NPOC mixing model used mean river conditions with maximum NPOC and maximum Cl − within groundwater, whereas the other mixing model used mean river conditions with minimum NPOC and minimum Cl − within groundwater. This approach was taken because of uncertainty in the source of groundwater sampled in the hyporheic zone. To evaluate potential drivers of organic carbon composition we correlated the pairwise Sorensen dissimilarity estimates with changes in NPOC concentration and changes in groundwater–surface water mixing conditions as estimated by changes in Cl − concentration. The statistical significance of the resulting relationships were evaluated with permutation-based Mantel tests (1,000 permuations) using the mantel function in the ecodist package. In addition, the median m / z value was found for each sample and distributions of these estimates were examined within each of the three water types studied here: river water, groundwater and hyporheic zone water. To determine whether observed changes in the m / z distributions were statistically significant, a Kruskal–Wallis test and its associated post-hoc test were used (functions kruskal.test and kruskalmc from the pgirmess library). These same statistical tests were used to evaluate shifts in POC across the three types of water. Ordinary least squares regression was used to evaluate whether OTU richness was related to groundwater–surface water mixing conditions, NPOC concentrations or POC concentrations; analogous analyses were carried out with suspended cell density as the dependent variable. Distance matrix regression and permutation-based Mantel tests were used to evaluate relationships between each of the three microbial community turnover metrics and changes in either NPOC concentration or mixing conditions. For each microbial community, we also calculated its median βNTI value based on its pairwise comparisons to all other sampled communities. For example, if community A was compared (separately) with communities B, C and D, there would be three separate βNTI estimates associated with community A; we found the median of these βNTI values. Each community, therefore, is associated with one median βNTI estimate; these estimates were related to the NPOC mixing model deviations by linear regression. The median βNTI estimates were also pooled into two groups—negative deviation or no deviation from the NPOC mixing model—and the resulting distributions were compared with a Kruskal–Wallis test. To identify OTUs potentially involved in the consumption of NPOC, microbial community composition was compared between pairs of hyporheic zone samples, which both deviated from the NPOC mixing model and which exhibited similar Cl − (±0.5 mg l −1 ) concentrations (that is, compared samples had similar groundwater–surface water mixing conditions, but different levels of deviation from the NPOC mixing model). Six pairs of samples were identified that met these criteria. Only OTUs with >1% relative abundance in at least one sample were used for this analysis. Taxonomic information was retrieved for OTUs showing an increase in relative abundance of >1% in the sample with the larger (that is, more negative) deviation from the NPOC mixing model. How to cite this article: Stegen, J. C. et al . Groundwater–surface water mixing shifts ecological assembly processes and stimulates organic carbon turnover. Nat. Commun. 7:11237 doi: 10.1038/ncomms11237 (2016).